An essential role for the N-terminal fragment of Toll-like receptor 9 in DNA sensing Toll-like receptor 9 (TLR9) is an innate immune sensor for microbial DNA that erroneously responds to self DNA in autoimmune disease. To prevent autoimmune responses, Toll-like receptor 9 is excluded from the cell surface and silenced until the N-terminal half of the ectodomain (TLR9N) is cleaved off in the endolysosome. Truncated Toll-like receptor 9 (TLR9C) senses ingested microbial DNA, although the precise role of the truncation remains controversial. Here we show that TLR9 is expressed on the surface of splenic dendritic cells. Following the cleavage of TLR9 in the endolysosome, N-terminal half of the ectodomain remains associated with truncated TLR9, forming the complex TLR9N+C. The TLR9-dependent cytokine production by Tlr9 −/− dendritic cells is rescued by a combination of TLR9N and TLR9C, but not by TLR9C alone. These results demonstrate that the TLR9N+C complex is a bona fide DNA sensor. Toll-like receptors (TLRs) sense a variety of microbial products. Cell-surface TLRs, including TLR4/MD-2, TLR1/TLR2 and TLR6/TLR2, recognize microbial membrane lipids, whereas TLR3, TLR7, TLR8 and TLR9 localize to intracellular organelles and recognize microbial nucleic acids [1] , [2] , [3] . Self/pathogen discrimination by DNA-sensing TLR9 was initially considered to depend on structural differences between self and microbial DNA, such as unmethylated CpG motifs [4] . However, despite its structure-dependent discrimination, TLR9 still has a risk of responding to self DNA [5] . Self/pathogen discrimination by TLR9 is therefore error prone and needs to be strengthened by endosomal DNA sensing-based mechanisms. While self-derived DNA is rapidly degraded by DNase, microbial DNA is resistant to degradation because it is encased in bacterial cell walls or viral particles. Microbial DNA is therefore able to reach endolysosomes and to stimulate TLR9 [6] (ref.6). The aberrant transportation of self DNA to endolysosomes has been shown to exacerbate autoimmunity [5] , [7] , [8] . In autoimmune diseases such as systemic lupus erythematosus or psoriasis, self DNA is complexed with autoantibodies or the cationic antimicrobial peptide LL37. These complexes are resistant to DNase and are delivered into endosomal compartments via FcR-mediated endocytosis, where they are able to activate TLR9, leading to dendritic cell (DC) activation and the production of type I interferon (IFN-I) [7] , [9] , [10] . In addition to ligand transportation, sensor transportation is also tightly controlled to prevent autoimmunity. TLR9 is reported to be localized mostly to the endoplasmic reticulum (ER) and transported to endolysosomes upon activation [11] , [12] . If TLR9 is forced to be expressed on the cell surface, TLR9 signals extracellular self DNA, leading to systemic lethal inflammation [13] . TLR9 sequestration from the cell surface is the second mechanism limiting TLR9 activation by self DNA. A third mechanism depends on the proteolytic cleavage of TLR9 (refs 14 , 15 ). After exiting the ER, the TLR9 ectodomain is cleaved by asparagine endopeptidase and/or cathepsins [16] , [17] . Truncated TLR9 (TLR9C), but not full-length (TLR9F), recruits MyD88. The precise role of proteolytic cleavage in DNA sensing is, however, still not clearly understood. TLR9F is able to sense DNA when its expression on the cell surface is forced by a mutation in the transmembrane domain [13] . Although these mechanisms that restrict TLR9 response to self DNA have been characterized, little is known about the expression, distribution and processing of endogenous TLR9. In the present study, we investigate these issues with newly established TLR9 monoclonal antibodies (mAbs). TLR9 is unexpectedly detected on the surfaces of splenic DCs but not on bone marrow-derived DCs (BMDCs) or B cells. The TLR9 in DCs is mostly cleaved, but the cleaved N-terminal fragment of the TLR9 ectodomain (TLR9N) remains associated with truncated TLR9 (TLR9C). TLR9C alone fails to sense DNA and requires TLR9N for signalling in response to DNA. These results demonstrate that TLR9N+C is a bona fide DNA sensor. Establishment of TLR9N- and TLR9C-specific mAbs To study endogenous TLR9, we established three mAbs to mouse TLR9. The specificities of the mAbs were verified by staining membrane permeabilized Ba/F3 cells expressing TLR3, 7, 8 and 9. Anti-mouse TLR9 specifically reacted with mouse TLR9 but did not cross-react with human TLR9 ( Fig. 1a ). Because the proteolytic cleavage of the TLR9 ectodomain has a role in DNA sensing, it was important to determine whether the epitopes for these mAbs were in TLR9N or TLR9C. We first identified the cleavage sites within TLR9. TLR9-GFP expressed in M12 B cell lymphoma was compared with that in PRAT4A-silenced M12 cells. PRAT4A is a TLR-specific chaperone [18] , and TLR9 fails to exit the ER and therefore remains unprocessed in the absence of PRAT4A. The fragment missing in PRAT4A-silenced M12 cells is therefore likely to be TLR9C ( Fig. 1b ). The identified TLR9C fragment was purified, and its N-terminal amino-acid sequence was determined. TLR9C was found to start at 461T or 467F ( Fig. 1c ). The determined cleavage sites were in the loop region between leucine-rich repeat 14 (LRR14) and LRR15 ( Fig. 1d ), consistent with the predictions from previous reports [15] , [17] . The presence of two distinct N-terminal fragments of TLR9C might be explained by stepwise processing of TLR9 by asparagine endopeptidase and cathepsins [16] . According to the N-terminal amino-acid sequences, a chimeric protein consisting of a signal peptide, N-terminal HA epitope, TLR9 ectodomain and transmembrane portion was expressed in Ba/F3 cells. Established cells were stained with anti-TLR9 mAb. Two mAbs, J15A7 and B33A4, reacted with TLR9N, whereas another mAb, C34A1, bound to TLR9C ( Fig. 1e ). J15A7 bound to TLR9N much less strongly than did B33A4. 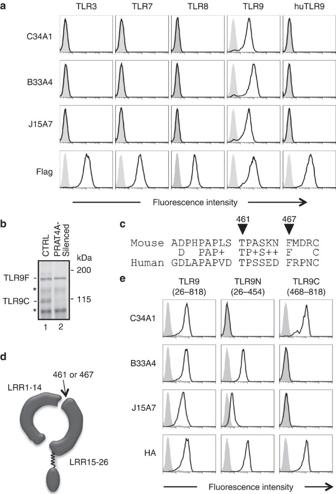Figure 1: Establishment of anti-mouse TLR9 mAbs. (a) Membrane-permeabilized Ba/F3 cells expressing mouse TLR3, 7, 8, 9 or human TLR9 were stained with anti-TLR9 or anti-FLAG antibodies as indicated. TLRs were tagged with the FLAG epitope at the C terminus. (b) TLR9-GFP was expressed in a B-cell lymphoma line M12 (lane 1) or PRAT4A-silenced M12 (lane 2), immunoprecipitated and immunoprobed with anti-GFP. Full-length (TLR9F) and truncated TLR9 (TLR9C) are indicated. Nonspecific bands are indicated by asterisks. (c) The first amino acids of the TLR9C isoforms, as determined by N-terminal amino-acid sequencing, are indicated by arrowheads. The human TLR9 amino-acid sequence is also shown. (d) Schematic representation of the cleavage sites in the TLR9 ectodomain. LRR, leucine-rich repeats. (e) Ba/F3 cells expressing the HA epitope, TLR9 ectodomain (TLR9 (26–818), TLR9N (26–454) or TLR9C (468–818)) and transmembrane region were established. These cells were membrane permeabilized and stained with anti-TLR9 or -HA antibodies. The grey histograms represent cells that stained with the second reagent alone. These experiments were repeated three times, and representative data are shown. Figure 1: Establishment of anti-mouse TLR9 mAbs. ( a ) Membrane-permeabilized Ba/F3 cells expressing mouse TLR3, 7, 8, 9 or human TLR9 were stained with anti-TLR9 or anti-FLAG antibodies as indicated. TLRs were tagged with the FLAG epitope at the C terminus. ( b ) TLR9-GFP was expressed in a B-cell lymphoma line M12 (lane 1) or PRAT4A-silenced M12 (lane 2), immunoprecipitated and immunoprobed with anti-GFP. Full-length (TLR9F) and truncated TLR9 (TLR9C) are indicated. Nonspecific bands are indicated by asterisks. ( c ) The first amino acids of the TLR9C isoforms, as determined by N-terminal amino-acid sequencing, are indicated by arrowheads. The human TLR9 amino-acid sequence is also shown. ( d ) Schematic representation of the cleavage sites in the TLR9 ectodomain. LRR, leucine-rich repeats. ( e ) Ba/F3 cells expressing the HA epitope, TLR9 ectodomain (TLR9 (26–818), TLR9N (26–454) or TLR9C (468–818)) and transmembrane region were established. These cells were membrane permeabilized and stained with anti-TLR9 or -HA antibodies. The grey histograms represent cells that stained with the second reagent alone. These experiments were repeated three times, and representative data are shown. Full size image TLR9 is expressed on the surface of splenic DCs TLR9 is believed to be sequestered from the cell surface, but endogenous TLR9 expression on the surface of primary immune cells has never been reported. Using the anti-TLR9 mAb, we next addressed the cell surface expression of TLR9. We first studied overexpressed TLR9 in Ba/F3 cells. As expected, cell-surface TLR9 was not detected on TLR9-expressing Ba/F3 cells, although the TLR9 mAbs did detect endosomal TLR9 in membrane permeabilized cells ( Fig. 2a ). Unc93B1 transports TLR9 from the ER to endolysosomes [11] . Unc93B1 may also have a role in transporting TLR9 to the cell surface. Unc93B1 was therefore overexpressed in Ba/F3 cells expressing TLR9. Both J15A7 and C34A1, but not the other anti-TLR9N, B33A4, detected cell surface TLR9 ( Fig. 2b ). J15A7 also detected cell surface TLR9 on splenic pDCs, CD8α + cDCs, CD4 + cDCs and double-negative cDCs ( Fig. 2c ). The specificity of the J15A7 staining was verified in Tlr9 −/− DCs. Cell surface TLR9 was not detected on splenic DCs from Unc93b1 3d/3d mice harbouring a loss-of-function mutation in the Unc93b1 gene [19] . Taken together with the finding that Unc93B1 overexpression induced the cell surface expression of TLR9 on Ba/F3 cells ( Fig. 2b ), these data suggest that Unc93B1 has an important role in transporting TLR9 to the cell surface. 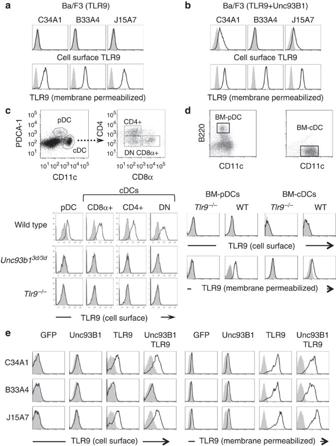Figure 2: TLR9 is expressed on the surface of splenic DCs. Ba/F3 cells expressing TLR9 alone (a) or TLR9 and Unc93B1 (b) were stained with the three anti-TLR9 antibodies. The upper panels show cell surface staining, whereas the lower panels show staining after membrane permeabilization. (c) Splenic cells from wild type,Unc93b13d/3dorTlr9−/−mice were stained with anti-TLR9 J15A7 together with mAbs against the indicated DC markers. The grey histograms represent cells that were not stained with the anti-TLR9 mAb. (d) BM-pDCs and BM-cDCs were stained with CD11c and B220 (BM-pDC) or CD11c (BM-cDCs) and anti-TLR9 J15A7. Open histograms show the proportion of CD11c and B220 (BM-pDCs) or CD11c (BM-cDCs)-gated cells that expressed TLR9. The upper panels show cell surface staining, whereas the lower panels show staining after membrane permeabilization. Grey histograms represent cells that did not exhibit anti-TLR9 staining. These experiments were repeated twice, and representative data are shown. (e) BM-cDCs were transduced with retroviral vectors encoding GFP, Unc93B1-mCherry or TLR9-GFP. BM-cDCs were subjected to cell surface staining or membrane permeabilization and staining with anti-TLR9 mAbs. Grey histograms represent cells that were not stained with anti-TLR9. Figure 2: TLR9 is expressed on the surface of splenic DCs. Ba/F3 cells expressing TLR9 alone ( a ) or TLR9 and Unc93B1 ( b ) were stained with the three anti-TLR9 antibodies. The upper panels show cell surface staining, whereas the lower panels show staining after membrane permeabilization. ( c ) Splenic cells from wild type, Unc93b1 3d/3d or Tlr9 −/− mice were stained with anti-TLR9 J15A7 together with mAbs against the indicated DC markers. The grey histograms represent cells that were not stained with the anti-TLR9 mAb. ( d ) BM-pDCs and BM-cDCs were stained with CD11c and B220 (BM-pDC) or CD11c (BM-cDCs) and anti-TLR9 J15A7. Open histograms show the proportion of CD11c and B220 (BM-pDCs) or CD11c (BM-cDCs)-gated cells that expressed TLR9. The upper panels show cell surface staining, whereas the lower panels show staining after membrane permeabilization. Grey histograms represent cells that did not exhibit anti-TLR9 staining. These experiments were repeated twice, and representative data are shown. ( e ) BM-cDCs were transduced with retroviral vectors encoding GFP, Unc93B1-mCherry or TLR9-GFP. BM-cDCs were subjected to cell surface staining or membrane permeabilization and staining with anti-TLR9 mAbs. Grey histograms represent cells that were not stained with anti-TLR9. Full size image In contrast to splenic DCs, BM-pDCs and BM-cDCs did not display easily detectable TLR9 on their cell surfaces ( Fig. 2d ). To gain insight into the mechanism controlling the cell surface expression of TLR9 on DCs, BM-cDCs were transduced with retroviral vectors encoding TLR9 or Unc93B1. The overexpression of TLR9, but not Unc93B1, enabled the detection of cell surface TLR9 on BM-cDCs ( Fig. 2e ). The coexpression of Unc93B1 weakly enhanced the cell surface expression of TLR9. The cell surface expression of TLR9 was positively correlated with the amount of TLR9. B33A4, an anti-TLR9N mAb, detected endosomal TLR9 but not cell surface TLR9 on BM-cDCs. Splenic B cells, monocytes and neutrophils were also stained with the anti-TLR9N mAb J15A7. Cell surface TLR9 was barely detectable on these cells ( Supplementary Fig. S1 ). TLR9 is reported to be expressed on the apical surface of intestinal epithelial cells (IEC) and to have a role in regulating colonic inflammation [20] . IECs were isolated from the mouse gut, and the cell surface expression of TLR9 on IECs was studied. TLR9 was undetectable on IECs ( Supplementary Fig. S2 ). In the cells studied, cell surface TLR9 was restricted to splenic DCs. TLR9N remains associated with TLR9C in endolysosomes TLR9N is thought to be cleaved off in endolysosomes [14] , [16] . Little is known about whether cleaved TLR9N is secreted, degraded or remains in endosomes. To address this issue, confocal microscopy was used to examine BM-pDCs stained with anti-TLR9N or -TLR9C antibodies. Calnexin staining was used to visualize the ER. Anti-TLR9N detected TLR9 mostly outside the ER, and its staining pattern showed no apparent difference from that of anti-TLR9C ( Fig. 3a ). Statistical analysis using ZEN confocal software (Carl Zeiss Microscopy) showed little significant colocalization of TLR9 with the ER. We next studied Unc93b1 3d/3d BM-pDCs, in which all the TLR9 remains uncleaved (TLR9F) in ER [11] . If TLR9 outside the ER is processed, and cleaved TLR9N is secreted or degraded, then anti-TLR9N should show much stronger staining in Unc93b1 3d/3d BM-pDCs than in wild-type BM-pDCs. Despite this expectation, two anti-TLR9N mAbs were able to detect as much TLR9 in wild-type BM-pDCs as in Unc93b1 3d/3d BM-pDCs ( Fig. 3b ). Moreover, when TLR9N was immunoprecipitated from supernatants of Ba/F3 cells expressing TLR9 or TLR9N alone, no secreted TLR9N was detectable ( Supplementary Fig. S3 ). These results suggest that TLR9N remained intact in endolysosomes after proteolytic cleavage. 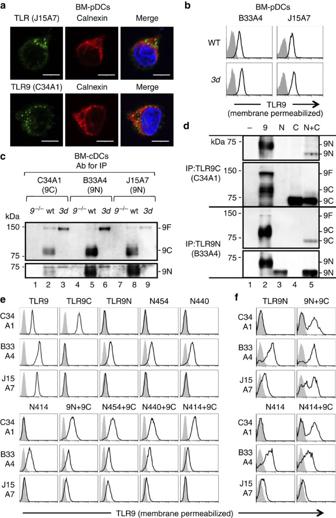Figure 3: TLR9N remains associated with TLR9C in endolysosomes. (a) BM-pDCs were stained with anti-TLR9N J15A7 or -TLR9C C34A1. Cells were counterstained with anti-Calnexin to locate the ER. Merged images are also shown. Scale bar, 5 μm. (b) BM-pDCs from wild type andUnc93b13d/3dmice were subjected to membrane permeabilization and staining with anti-TLR9 as indicated. Grey histograms represent cells that stained with the second reagent alone. (c) BM-cDCs from wild type,Unc93b13d/3dandTlr9−/−mice were subjected to immunoprecipitation with the indicated mAbs and immunoprobing with anti-TLR9N or anti-TLR9C antibodies. (d) TLR9, TLR9N truncated at 466 (TLR9N) or TLR9 lacking the TLR9N region from 36–466 (TLR9C) were expressed in Ba/F3 cells expressing Cathepsin L, Unc93B1 and the NF-κB–GFP reporter construct as indicated. These cells were subjected to immunoprecipitation with anti-TLR9N or anti-TLR9C and immunoprobing. (e) TLR9, TLR9 lacking 36–466 (TLR9C), and TLR9 truncated at 466, 454, 440 or 414 (N466, N454, N440 or N414) were expressed in Ba/F3 cells expressing cathepsin L, Unc93B1 and NF-κB–GFP, as indicated. These Ba/F3 cells were subjected to membrane permeabilization and staining with the indicated anti-TLR9 mAbs. These experiments were repeated at least twice. (f) BM-cDCs were transduced with TLR9N (N466) or N414 with or without TLR9C. These cells were then stained with anti-TLR9N mAbs. The grey histograms represent cells that were not stained with anti-TLR9. These experiments were repeated twice, and representative data are shown. Figure 3: TLR9N remains associated with TLR9C in endolysosomes. ( a ) BM-pDCs were stained with anti-TLR9N J15A7 or -TLR9C C34A1. Cells were counterstained with anti-Calnexin to locate the ER. Merged images are also shown. Scale bar, 5 μm. ( b ) BM-pDCs from wild type and Unc93b1 3d/3d mice were subjected to membrane permeabilization and staining with anti-TLR9 as indicated. Grey histograms represent cells that stained with the second reagent alone. ( c ) BM-cDCs from wild type, Unc93b1 3d/3d and Tlr9 −/− mice were subjected to immunoprecipitation with the indicated mAbs and immunoprobing with anti-TLR9N or anti-TLR9C antibodies. ( d ) TLR9, TLR9N truncated at 466 (TLR9N) or TLR9 lacking the TLR9N region from 36–466 (TLR9C) were expressed in Ba/F3 cells expressing Cathepsin L, Unc93B1 and the NF-κB–GFP reporter construct as indicated. These cells were subjected to immunoprecipitation with anti-TLR9N or anti-TLR9C and immunoprobing. ( e ) TLR9, TLR9 lacking 36–466 (TLR9C), and TLR9 truncated at 466, 454, 440 or 414 (N466, N454, N440 or N414) were expressed in Ba/F3 cells expressing cathepsin L, Unc93B1 and NF-κB–GFP, as indicated. These Ba/F3 cells were subjected to membrane permeabilization and staining with the indicated anti-TLR9 mAbs. These experiments were repeated at least twice. ( f ) BM-cDCs were transduced with TLR9N (N466) or N414 with or without TLR9C. These cells were then stained with anti-TLR9N mAbs. The grey histograms represent cells that were not stained with anti-TLR9. These experiments were repeated twice, and representative data are shown. Full size image We next asked whether TLR9N is associated with another molecule in endosomes. TLR9N is reported to coprecipitate with TLR9F or TLR9C in the RAW264.7 macrophage cell line [15] , suggesting that TLR9N physically associates with TLR9C or TLR9F. To confirm this finding with endogenous TLR9 in primary immune cells, anti-TLR9C was used to immunoprecipitate TLR9F or TLR9C from BM-cDCs. Appreciable amounts of TLR9N coprecipitated with both TLR9C and TLR9F ( Fig. 3c , lane 2). Similarly, TLR9C was coprecipitated by two anti-TLR9N antibodies ( Fig. 3c , lane 5 and 8). As a majority of TLR9 is processed in BM-cDCs ( Fig. 3c ), TLR9C and TLR9N are likely to be associated with each other rather than with TLR9F. To completely exclude the involvement of TLR9F, TLR9N truncated at 466 and TLR9C beginning at 467 were expressed in Ba/F3 cells, which do not express detectable levels of endogenous TLR9 [21] (ref.21). TLR9N and TLR9C both migrated much more rapidly in SDS–polyacrylamide gel electrophoresis (SDS–PAGE) than TLR9N or TLR9C processed from TLR9F ( Fig. 3d , compare lane 2 with lane 3 for TLR9N or with lane 4 for TLR9C), most likely due to defects in glycosylation. The faster migration in SDS–PAGE was not altered by the coexpression of the other fragment, TLR9N or TLR9C ( Fig. 3d , compare lane 3 with lane 5 for TLR9N or lane 4 with lane 5 for TLR9C). When TLR9C and TLR9N were immunoprecipitated, the other fragments were weakly but appreciably coprecipitated ( Fig. 3d , lane 5). These results demonstrate a direct association between TLR9N and TLR9C. The C-terminal LRR of TLR9N mediates its binding to TLR9C Extra amino-acid residues between LRR14 and LRR15 (441-470) are predicted to form a loop protruding from the LRRs that contains the cleavage site [22] . Consistent with this model, TLR9C began at 461T or 467F, both of which are close to the end of the loop and the beginning of LRR15. To investigate the role of these extra amino acids in TLR9N in its interaction with TLR9C, TLR9Ns truncated at 440 or 454 were expressed in Ba/F3 cells, and the cells were then stained with TLR9 mAbs. B33A4 bound to TLR9N (N466), either alone or with TLR9C ( Fig. 3e ). The staining pattern of J15A7 was distinct from that of B33A4. Whereas J15A7 and B33A4 exhibit comparable levels of binding to full-length TLR9-expressing cells, J15A7 binds to TLR9N-expressing cells much less strongly than does B33A4. When TLR9C was co-expressed with TLR9N, however, J15A7 binding was comparable to that of B33A4 ( Fig. 3e ). This suggests that J15A7 is likely to react preferentially with the TLR9N+C complex over TLR9N alone, most likely due to a conformational change induced in TLR9N in the absence of TLR9C. The truncation of TLR9N at 454 or 440 did not alter B33A4 staining or the TLR9C-dependent augmentation of J15A7 binding to TLR9N ( Fig. 3e ), suggesting that the extra amino acids in TLR9N are not directly involved in assembling TLR9N+C. The tandem repeats of the leucine-rich motif (LRM) are stabilized by hydrogen bonds between adjacent LRMs [22] . The interaction between TLR9N and TLR9C may depend on hydrogen bonds between LRR14 and LRR15. To address this possibility, TLR9N lacking LRR14, that is, TLR9N truncated at 414 (N414), was studied. N414 was detected by B33A4, demonstrating that the global structure of TLR9N is not altered by the truncation. J15A7 only weakly detected N414 alone, and the coexpression of TLR9C failed to augment J15A7 staining ( Fig. 3e ). To exclude the possibility that J15A7 does not interact with N414 alone, N414 was expressed as a fusion protein, as shown in Fig. 1e , and stained by J15A7. In the context of the fusion, J15A7 interacted with N414 as strongly as it did with N454 ( Supplementary Fig. S4 ). Further, N414 was expressed in BM-cDCs with or without TLR9C. J15A7 bound to N414 weakly but appreciably, similar to its binding to TLR9N (N466), but the binding was not augmented by TLR9C coexpression ( Fig. 3f ). These results strongly suggest that LRR14 is required for the interaction of TLR9N with TLR9C. TLR9N is required for DNA sensing The role of TLR9N in TLR9 signalling was then studied. Previous studies have demonstrated that TLR9C alone is able to bind to its ligand and recruit the signalling adaptor MyD88 (refs 14 , 15 ). TLR9F, in contrast, is able to bind to DNA but unable to recruit MyD88 (ref. 14 ). The association of TLR9N with TLR9C led us to examine the role of TLR9N in TLR9C signalling. TLR9 and MyD88 were overexpressed in M12 B cells. Anti-TLR9N or -TLR9C antibodies were used for immunoprecipitation, and the coprecipitation of MyD88 was examined. Anti-TLR9N and anti-TLR9C both coprecipitated MyD88, and the degree of coprecipitation increased with CpG-B stimulation ( Fig. 4a ). MyD88 coprecipitation with anti-TLR9N demonstrated that MyD88 was recruited to either TLR9F or TLR9N+C. If TLR9F is unable to recruit MyD88 [14] (ref.14), then TLR9N+C is likely to induce signalling in response to DNA. To exclude the involvement of TLR9F, we studied Ba/F3 cells expressing TLR9N, TLR9C or both. These cells also expressed a reporter construct that drives the expression of green fluorescent protein (GFP) in response to NF-κB activation. The cells were stimulated with CpG-B, and GFP induction was measured. Ba/F3 cells expressing TLR9C alone failed to reproduce DNA sensing by TLR9C [15] . GFP was induced only when TLR9N was co-expressed with TLR9C ( Fig. 4b ). The requirement for the loop between LRR14 and LRR15 was next investigated using TLR9N truncated at 440 or 454. TLR9 responses were not impaired by TLR9N truncation to 440 ( Fig. 4b ). Thus, the loop between LRR14 and LRR15 is not required for TLR9-dependent NF-κB activation. In contrast, TLR9N lacking LRR14 (N414) failed to confer DNA-dependent NF-κB activation in the presence of TLR9C, demonstrating a correlation between TLR9N+C complex formation ( Fig. 3e ) and TLR9 response. 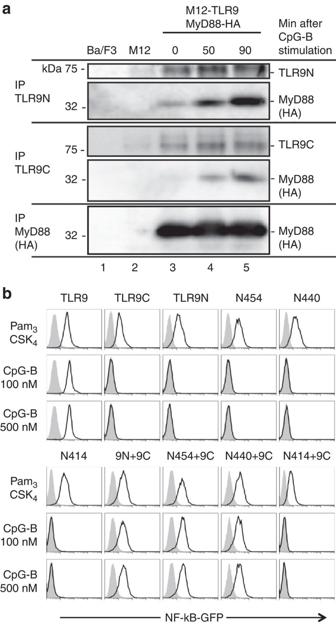Figure 4: TLR9N is required for signalling in response to DNA. (a) M12 B cells expressing TLR9 and MyD88-HA were stimulated with CpG-B (0.9 μM) and subjected to immunoprecipitation with anti-TLR9N B33A4, -TLR9C C34A1 or -HA and immunoprobing with anti-TLR9C or anti-TLR9N, as indicated. An unrelated cell line (Ba/F3) and plain M12 were used as negative controls. (b) The Ba/F3 cells shown inFig. 3ewere left unstimulated or stimulated for 24 h with 100 nM, 500 nM CpG-B or 1 μg ml−1Pam3CSK4as indicated. The level of GFP induction was determined by flow cytometry. These experiments were repeated twice, and representative data are shown. Figure 4: TLR9N is required for signalling in response to DNA. ( a ) M12 B cells expressing TLR9 and MyD88-HA were stimulated with CpG-B (0.9 μM) and subjected to immunoprecipitation with anti-TLR9N B33A4, -TLR9C C34A1 or -HA and immunoprobing with anti-TLR9C or anti-TLR9N, as indicated. An unrelated cell line (Ba/F3) and plain M12 were used as negative controls. ( b ) The Ba/F3 cells shown in Fig. 3e were left unstimulated or stimulated for 24 h with 100 nM, 500 nM CpG-B or 1 μg ml −1 Pam 3 CSK 4 as indicated. The level of GFP induction was determined by flow cytometry. These experiments were repeated twice, and representative data are shown. Full size image To further study the responses of TLR9N+C, Tlr9 −/− BM-cDCs were transduced with retroviral vectors encoding TLR9, TLR9N, TLR9C or TLR9N+TLR9C. TLR9 expression was confirmed by staining membrane-permeabilized cells with the anti-TLR9 mAb ( Fig. 5a ). TLR9F and TLR9C were expressed in over 80% of the Tlr9 −/− BM-cDCs. The expression of TLR9N+C was estimated based on the TLR9C-dependent augmentation of J15A7 binding to TLR9N. More than 50% of cells were considered J15A7 high . These BM-cDCs were stimulated with lipid A, CpG-A or CpG-B, and the resulting levels of IL-12p40, TNFα, and IFNβ were determined by ELISA. Complementation with TLR9N+C was able to induce all the cytokines studied to the same degree observed for TLR9 ( Fig. 5b ), demonstrating that TLR9N+C is a DNA-sensing complex. 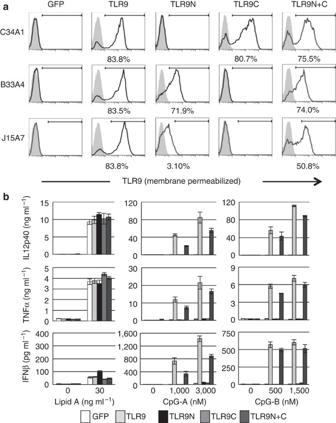Figure 5: TLR9N+C is able to complement TLR9-dependent cytokine production inTlr9−/−BM-cDCs. (a)Tlr9−/−BM-cDCs were transduced with a retroviral vector encoding GFP as a negative control, TLR9, TLR9N (N466), TLR9C or TLR9N+C. BM-cDCs were subjected to membrane permeabilization and staining with anti-TLR9 mAbs. Grey histograms indicate the cells that were stained by the second reagent alone. The gates for positivity and the positive percentages are also shown. The gate for J15A7 was considered to represent TLR9N+C cells. (b) BM-cDCs were stimulated with lipid A or TLR9 ligands, and the production of the indicated cytokines was determined by ELISA. The values show the averages and s.d. from triplicate experiments (wells). The experiments were repeated twice, with the same results. Figure 5: TLR9N+C is able to complement TLR9-dependent cytokine production in Tlr9 −/− BM-cDCs. ( a ) Tlr9 −/− BM-cDCs were transduced with a retroviral vector encoding GFP as a negative control, TLR9, TLR9N (N466), TLR9C or TLR9N+C. BM-cDCs were subjected to membrane permeabilization and staining with anti-TLR9 mAbs. Grey histograms indicate the cells that were stained by the second reagent alone. The gates for positivity and the positive percentages are also shown. The gate for J15A7 was considered to represent TLR9N+C cells. ( b ) BM-cDCs were stimulated with lipid A or TLR9 ligands, and the production of the indicated cytokines was determined by ELISA. The values show the averages and s.d. from triplicate experiments (wells). The experiments were repeated twice, with the same results. Full size image The newly established mAbs to TLR9N or TLR9C have been used to identify TLR9N+C as a bona fide DNA-sensing form of TLR9. TLR9 that is overexpressed is reported to be completely cleaved in the phagosome [14] . Here, the majority of endogenous TLR9 in the steady-state DCs is shown to be processed and to reside outside the ER. A previous report showed that TLR9N is associated with TLR9C or TLR9F in a macrophage cell line [15] . Consistent with this observation, endogenous TLR9N in BM-cDCs remains associated with TLR9C. Although TLR9C alone is reported to respond to DNA, TLR9C requires TLR9N for DNA sensing. TLR9N+C is primarily responsible for the DNA-dependent TLR9 responses observed in DCs. A previous study using deletion mutations at TLR9N suggested that TLR9N is required for interaction with DNA and subsequent TLR9 activation [23] . In the present study, we employ another approach, a complementation strategy, and similarly conclude that TLR9N is required for TLR9 responses. Even when TLR9N and TLR9C are independently produced in the ER, they are able to self-assemble. TLR9N+C is able to activate an NF-κB reporter in the Ba/F3 cell line and to induce the expression of a variety of cytokines, including TNFα, IL-12p40 and IFNβ, in Tlr9 −/− BM-cDCs. Considering that IRF7 activation is required for IFNβ production [24] , these findings show that TLR9N+C is able to activate IRF7-dependent signalling pathways as well as NF-κB-dependent pathways. Although TLR9C alone is reported to interact with DNA [14] , [15] , this interaction, if it occurs, does not activate downstream signalling pathways in our experimental systems. The DNA ligand induces an allosteric change in the cytoplasmic signalling domain of the preformed TLR9 dimer [25] . The interaction of DNA with TLR9C alone may not be sufficient to induce this allosteric change. TLR ectodomains consist of the tandem repeats of LRM, which is typically 24 amino acids in length [22] . The LRM adopts a loop structure, beginning with a short β-strand followed by a β-turn. Tandem repeats of LRM form a solenoid structure with parallel β-sheets. Consecutive β-sheets and β-turns form a continuous hydrogen-bonded, packed structure, generating a curved solenoid with the β-sheets on the concave side. TLR ectodomains are stabilized by their interior hydrophobic cores and hydrogen bonds between adjacent β-sheets [22] . The LRRs of the TLR ectodomains, especially those of TLR7, 8 and 9, are longer than 24 amino acids. The extra residues form a loop that protrudes from the convex or planar side of the LRR solenoid. A tentative loop is thought to be located between LRR14 and LRR15 in the TLR9 ectodomain and is predicted to be cleaved [15] . Consistent with this prediction, the present study shows that TLR9C begins at the C-terminal end of the loop. Considering that the protruding loop does not contribute to either the inner hydrophobic bonds or the hydrogen bonds between β-sheets, the proteolysis of the loop is not likely to influence the basic solenoid structure. The association between TLR9N and TLR9C is likely to be mediated by the hydrogen bonds between the β-sheets of LRR14 and LRR15, not by the loop between LRR14 and LRR15. This hypothesis is supported by the behaviours of the TLR9N mutants. A TLR9N construct lacking the loop (N440) is able to confer DNA-responsiveness to TLR9C, but TLR9N lacking LRR14 (N414) is not. J15A7 staining of TLR9N is amplified by TLR9C coexpression, suggesting that J15A7 preferentially binds to TLR9N+C over TLR9N alone. Amplification induced by TLR9C coexpression is observed for N440 but not N414, indicating that N414 fails to associate with TLR9C. Therefore, LRR14 is required for the interaction of TLR9N with TLR9C. Although TLR9N has been reported to be dispensable for the TLR9 response [14] , [15] , the present study shows that TLR9N is required for TLR9 responses. It is possible that uncleaved TLR9F is not competent for DNA sensing and that TLR9 proteolytic cleavage activates this activity. Uncleaved TLR9F is, however, reported to be activated in vivo when its expression on the cell surface is forced [13] . These results suggest that TLR9F is able to respond to DNA. The role of proteolytic cleavage in the TLR9 response remains unresolved but can be addressed by comparing TLR9 and TLR9N+C. Complementation with TLR9 generates both TLR9F and TLR9N+C, whereas complementation with TLR9N+TLR9C generates TLR9N+C only. A comparison of the cytokine production by BM-cDCs complemented with TLR9 and TLR9N+TLR9C reveals no significant differences. Future studies should focus on other cell types, such as B cells and pDCs. Another mechanism of TLR9 silencing, exclusion from cell surface, is found to be leaky in splenic DCs. Cell surface TLR9 is detected on splenic DCs but not BM-cDCs. Cell surface TLR9 is detectable on TLR9-overexpressing BM-cDCs but not Unc93B1-overexpressing cells. In BM-cDCs, TLR9 expression may not be sufficient for its cell surface expression. Considering that the forced expression of TLR9 on the cell surface causes lethal systemic inflammation [13] , cell surface TLR9 expression is likely to be silenced in splenic DCs. The TLR9N mAb J15A7 is able to detect cell surface TLR9 on splenic DCs in normal mice, whereas the other TLR9N mAb, B33A4, is not. Given that B33A4 mAb detects both TLR9F and TLR9N+C in endosomes, the failure of B33A4 mAb to detect cell surface TLR9 is unlikely to be due to the cleavage of the TLR9 ectodomain. Rather, cell surface TLR9 is likely to adopt a conformational state distinct from that of endosomal TLR9. This distinct conformation may be linked to TLR9 silencing on the cell surface. Further studies are needed to characterize the functional difference between cell surface and endosomal TLR9. Reagents and antibodies Pam 3 CSK 4 was purchased from EMC Microcollections. Lipid A Re:595 was purchased from Sigma-Aldrich. CpG-A 1585 (5′-G * G * GGTCAACGTTGAG * G * G * G * G * G-3′; asterisks represent phosphorothioated bases) was synthesized by Hokkaido System Science. CpG-B 1688 (5′-TCCATGACGTTCCTGATGCT-3′, all phosphorothioated) was synthesized by FASMAC. Recombinant mouse GM-CSF was purchased from R&D Systems. Recombinant murine Flt-3 ligand was purchased from PeproTech. Digitonin was purchased from Wako and Nacalai. The anti-FLAG antibody and puromycin were purchased from Sigma-Aldrich. G418 was purchased from Nacalai. Anti-HA antibody–conjugated beads and the anti-HA antibody (clone 3F10) were purchased from Roche. The rabbit anti-GFP polyclonal antibody (pAb) used for western blotting was purchased from Invitrogen, and the anti-GFP (FM264) mAb used for immunoprecipitation was previously generated in our laboratory [26] . For immunoprobing TLR9C, a rabbit pAb against the TIR domain was developed in our laboratory. For immunoprobing TLR9N, a rabbit pAb against amino acids 200–300 of mouse TLR9 (# ab13928) was purchased from Abcam. Plasmid constructs The C termini of mouse TLR3, 7, 8 and 9, human TLR9, Unc93B1 and Myd88 were tagged with FLAG-6xHis, HA or GFP epitopes as indicated in the figures. They were generated by PCR and cloned into retroviral pMX, pMXpuro or pMXneo vectors (kindly provided by Dr Kitamura, Tokyo, Japan). To suppress mouse PRAT4A expression in M12 cells, we also constructed the shRNA-expressing retroviral vector pSSCH, as described previously [26] . For the constructs encoding TLR9N fragments ( Figs 3 and 4 ), TLR9 fragments corresponding to amino acids 1–414 (TLR9N414), 1–440 (TLR9N440), 1–454 (TLR9N454), or 1–466 (TLR9N466) were cloned into the pMX vector. For the TLR9C constructs, TLR9 fragments corresponding to amino acids 1–35 (the signal peptide and following 10 amino acids) fused to amino acids 441–1,032 (441TLR9C), 455–1,032 (455TLR9C) or 467–1,032 (467TLR9C) were cloned into the pMX vector using the In-Fusion HD cloning kit (Clontech Laboratories, Inc.). Mice and cell lines C57BL/6 mice were purchased from Japan SLC, Inc. (Shizuoka, Japan). The Tlr9 −/− mice were kind gifts from Prof Shizuo Akira (Osaka University, Japan). The Unc93B1 3d/3d mice were kindly provided by Professor Bruce Beutler and the Scripps Research Institute. Mice were maintained in the animal facility of the Institute of Medical Science at the University of Tokyo and all studies using mice were approved by the Institutional Animal Care and Use Committee. Ba/F3 cells and M12 cells were cultured in Roswell Park Memorial Institute (RPMI) 1640 medium supplemented with 10% fetal bovine serum, 100 units per ml penicillin, 100 μg ml −1 streptomycin, 300 μg ml −1 glutamine and 50 μM 2-ME. IL-3 was added to the culture medium for the Ba/F3 cells. The construction of a Ba/F3 line with NF-κB-GFP (BaκB) was described previously 21 . Retroviral transduction The pMX, pMXpuro and pMXneo vectors were transfected into Plat-E packaging cells with FuGene6 (Roche). After 2 days of incubation, supernatants were obtained as virus suspensions. Cells were infected using a mixture of virus suspension and DOTAP (Roche). Induction of DCs and macrophages from BM cells BM-cDCs and BM-pDCs were prepared as described previously [21] . Briefly, BM cells were flushed from mouse tibiae and femurs. The red blood cells were lysed, and the remaining cells were cultured at 37 °C for 1 week in RPMI 1640 medium supplemented with 10% FCS, penicillin–streptomycin–glutamine and 50 mM 2-ME. Macrophage, cDC and pDC differentiation was induced by 100 ng ml −1 M-CSF, 10 ng ml −1 GM-CSF and 50 ng ml −1 Flt-3 ligand, respectively. Retroviral transduction of BMDCs BM cells from TLR9-deficient mice were cultured with 10 ng ml −1 of recombinant murine GM-CSF. After 3 days of culture, cells were seeded on 24-well tissue culture dishes at 5 × 10 5 cells per well in 150 μl of RPMI 1640 medium supplemented with 10% FCS. A 250-μl aliquot of retroviral suspension and 250 μl of medium were added to the BM cells with 15 ng ml −1 of recombinant murine GM-CSF and 6 μg ml −1 of DOTAP. For co-transduction with multiple vectors, 250 μl of each retrovirus suspension encoding two different truncated TLR9 were added to the BM cells as described above. Cells were centrifuged at 840 g for 60 min at room temperature. On the next day, 1 ml of medium supplemented with GM-CSF was added. The retrovirus transduction procedure was repeated on days 5 and 7, and fresh medium was added on the days following each transduction. On day 9, all media, including the retroviruses, were removed; the cells were washed three times; and fresh medium supplemented with GM-CSF was added. On day 10, the BMDCs were harvested and stimulated with TLR ligands. ELISA The cytokine and interferon levels in the culture supernatants were measured with ELISA kits (R&D Systems). TLR9 cleavage-site analysis GFP-tagged mouse TLR9 was stably expressed in M12 cell line. Aliquots of 1 × 10 10 cells were collected and prepared for immunoprecipitation in lysis buffer (150 mM NaCl, 50 mM Tris·HCl (pH 7.4), 0.5% Triton X-100, 10 μg ml −1 aprotinin, 10 μg ml −1 leupeptin, 1 mM PMSF). Anti-GFP agarose beads (MBL, Japan) were added to the lysate and incubated overnight at 4 °C. The beads were collected and washed four times in washing buffer (150 mM NaCl, 30 mM Tris·HCl (pH 7.4), 0.1% Triton X-100), and the precipitated protein was eluted in buffer (150 mM NaCl, 30 mM glycine·HCl (pH 2.5), 0.1% Triton X-100). The eluted sample was dialysed against a new buffer (10 mM NaCl, 0.1% Triton X-100) and concentrated by freeze drying. The concentrated sample was reconstructed in sample buffer (2% SDS, 10% glycerol, 62.5 mM Tris·HCl (pH 6.8), 0.025% bromophenol blue, 5% 2-ME) and subjected to SDS–PAGE. The separated protein was transferred to a PVDF membrane in CAPS transfer buffer. Transferred protein was visualized by Coomassie Blue, and the band corresponding to the C-terminal fragment of TLR9C was cut out. The TLR9C gel band was subjected to N-terminal amino-acid analysis, and the amino-acid sequence was detected by APRO Science Co., Ltd. (Japan). Confocal imaging BM-pDCs were stained with anti-CD11c-Pacific Blue and anti-B220-APC to enable the sorting of CD11c + B220 + DC cells with a FACSAria instrument. The sorted pDCs were allowed to adhere to coverslips overnight and were then fixed in 4% paraformaldehyde for 10 min and permeabilized with 0.1% Triton X-100 in 2.5% BSA Blocking One for 30 min. pDCs were incubated with anti-TLR9 and anti-Calnexin primary antibodies (Abcam) for 90 min at 37 °C, washed and then incubated with Alexa Fluor 488- or 568-conjugated secondary antibodies (Invitrogen) for 90 min at 37 °C. The immunostained pDCs were examined under an LSM710 confocal microscope with a × 63 NA1.4 Plan-Apochromat oil immersion lens (Carl Zeiss Microscopy). Fluorescent images were acquired and analysed using the LSM710 ZEN software. The colocalization of TLR9 with Calnexin was analysed using LSM710 ZEN according to the manual provided with the software. At least two independent measurements were conducted for each image. Pearson’s correlation coefficients were used for the statistical analysis of colocalization. The Pearson’s coefficients are shown as absolute values. A Pearson’s coefficient <0.2 represents poor colocalization. Anti-mouse TLR9 mAb To establish a mAb against mouse TLR9, BALB/c Tlr9 −/− mice were immunized with Ba/F3 cells expressing mouse TLR9 (Ba/F3_mTLR9). Four days after the final immunization, splenic cells were fused with SP2/O myeloma cells. Hybridomas that produced anti-mouse TLR9 mAbs were selected by flow cytometry staining of the Ba/F3 cells used for immunization. Three mAbs, J15A7 (IgG1/κ), C34A1 (IgG2a/κ) and B33A4 (IgG2a/κ), were isolated and used in the present study. We used these antibodies at the following concentrations: for cell surface staining: all antibodies 0.2 μg ml −1 ; for internal staining, J15A7: 0.2 μg ml −1 , C34A1: 0.075 μg ml −1 , B33A4: 0.075 μg ml −1 ; for confocal microscopy: all antibodies: 1 μg ml −1 . Cell staining For the staining of BM cells and splenocytes, cells were preincubated with anti-CD16/CD32 (clone: 93) and stained with fluorescein-conjugated antibodies specific to the following markers for flow cytometry analysis: CD4 (GK1.5), CD8α (53–6.7), CD11c (HL3), B220 (RA3-6B2) and PDCA-1 (927, 129c1). Single-cell splenocyte suspensions were prepared as described previously [27] . Cells were incubated at 4 °C with biotinylated mAbs diluted in staining buffer (1 × PBS with 2.5% fetal bovine serum and 0.1% NaN 3 ), followed by incubation with a streptavidin-conjugated antibody. For the internal staining, cells were permeabilized with 0.05% or 0.1% saponin (Sigma-Aldrich S5421 or WAKO 193-00162) in staining buffer; subsequent steps were performed in saponin buffer. Stained cells were analysed with FACSCalibur or FACSAria flow cytometers (BD Biosciences). Immunoprecipitation and western blotting Cells were washed and lysed in lysis buffer consisting of 1% digitonin, 20 mM Tris·HCl (pH 7.4), 150 mM NaCl, 1 mM CaCl 2 , 1 mM MgCl 2 , 10% glycerol, 1 mM DTT and Complete Protease Inhibitor Cocktail (Roche). After incubation on ice, the lysates were centrifuged, and the debris was removed. For immunoprecipitation, anti-HA matrix (Roche, clone 3F10) or N -hydroxysuccinimide-activated Sepharose 4FF beads coupled to the anti-mouse TLR9 mAb were added to the cell lysates and incubated at 4 °C. Then, the beads were washed three times with 0.1% digitonin, and the bound proteins were eluted by boiling in SDS sample buffer (125 mM Tris·HCl (pH 6.8), 20% glycerol, 4% SDS, 10% 2-ME, 0.005% bromophenol blue). After electrophoresis, samples were transferred to PVDF membranes and subjected to immunoblotting. Intestinal epithelial cells The intestines were opened longitudinally and washed extensively several times with ice-cold PBS. The intestinal tissue was then cut into 0.5-cm pieces and incubated in 1 mM EDTA/PBS at 37 °C for 20 min with gentle shaking. After passage through a 70-μm cell strainer, the cells were washed twice with DMEM containing 20% fetal calf serum (FCS). The isolated cells were stained with anti-EpCAM (eBioscience, clone G8.8), anti-CD45 (Biolegend, clone 30-F11) Abs and 7-aminoactinomycin D (7-AAD, BD). The 7-AAD − /CD45 − /EpCAM + cells were considered IECs and used for the further analysis of TLR9 expression. How to cite this article: Onji, M. et al . An essential role for the N-terminal fragment of Toll-like receptor 9 in DNA sensing. Nat. Commun. 4:1949 doi: 10.1038/ncomms2949 (2013).